Structure-based engineering of substrate specificity for pinoresinol-lariciresinol reductases Pinoresinol–lariciresinol reductases (PLRs) are enzymes involved in the lignan biosynthesis after the initial dimerization of two monolignols, and this represents the entry point for the synthesis of 8-8′ lignans and contributes greatly to their structural diversity. Of particular interest has been the determination of how differing substrate specificities are achieved with these enzymes. Here, we present crystal structures of Ii PLR1 from Isatis indigotica and pinoresinol reductases (PrRs) At PrR1 and At PrR2 from Arabidopsis thaliana , in the apo, substrate-bound and product-bound states. Each structure contains a head-to-tail homodimer, and the catalytic pocket comprises structural elements from both monomers. β4 loop covers the top of the pocket, and residue 98 from the loop governs catalytic specificity. The substrate specificities of Ii PLR1 and At PrR2 can be switched via structure-guided mutagenesis. Our study provides insight into the molecular mechanism underlying the substrate specificity of PLRs/PrRs and suggests an efficient strategy for the large-scale commercial production of the pharmaceutically valuable compound lariciresinol. Lignans are a major group of secondary metabolites in plants [1] . This family has numerous biological effects in humans (e.g., anticancer [2] , antiviral [3] , antioxidant [4] , and immunosuppression [5] ) owing to their structural diversity—nearly 2000 distinct lignans have been reported. For example, the furofuran lignans such as kandelisesquilignan A/B and terminaloside K have antioxidant effects [6] , [7] . The dibenzylbutyrolactone lignans including arctigenin, traxillagenin, arctiin, traxillaside, and their glycosides have neuroprotective activities [8] . Finally, the aryltetralin lignan podophyllotoxin [9] is the precursor for the semi-synthesis of anticancer drugs such as etoposide [10] . Lignans biosynthesis starts with the coupling of two coniferyl alcohols by an oxidase (laccase or peroxidase) with the aid of a dirigent protein to form pinoresinol [11] . Pinoresinol/lariciresinol reductase (PLR), an NADPH-dependent reductase, converts pinoresinol to lariciresinol and subsequently to secoisolariciresinol [12] . Because the reductive steps that give rise to lariciresinol and secoisolariciresinol represent entry points for the biosynthesis of the lignan subclasses furofurans, dibenzylbutane, dibenzylbutyrolactone, and aryltetrahydronaphthalene [13] , PLR is regarded as a pivotal enzyme that contributes to lignan structural diversity. Moreover, variation in both the composition and accumulation of lignans among different plant species, organs, and developmental stages can be ascribed, at least in part, to the characteristics of reactions catalyzed by PLRs as well as their expression patterns [14] . Therefore, characterization of the catalytic mechanisms of PLRs—especially their substrate selectivity—is particularly crucial for understanding the molecular basis of the remarkable diversity of both chemical structures and biological activities of lignans. The substrate selectivity of PLRs has attracted considerable attention [12] . Most PLRs that have been characterized reduce both pinoresinol and lariciresinol efficiently to produce lariciresinol and secoisolariciresinol, respectively [12] . Known exceptions are Arabidopsis thaliana reductases that have substrate preference for pinoresinol, but only weak ( At PrR1) or no activity ( At PrR2) toward lariciresinol and are thus named pinoresinol reductases (PrRs) [15] . A recent study indicated that the L174I mutant of Camellia sinensis PLR1 ( Cs PLR1) loses the capacity to reduce pinoresinol and specifically catalyzes the conversion of lariciresinol to secoisolariciresinol, but the underlying mechanism is unclear [16] . The three-dimensional structure of Thuja plicata PLR1 ( Tp PLR1) has been elucidated and indicates that K138 is responsible for the basic catalysis, because the mutant K138A lacks the ability to convert pinoresinol [17] . However, the apo structure does not provide sufficient information to interpret the substrate-selective mechanism of PLRs/PrRs. Phylogenetic analysis of PLRs/PrRs from different species has revealed that Isatis indigotica PLR1 ( Ii PLR1), a key enzyme involved in lariciresinol biosynthesis, has the closest relationship to At PrRs with a high level of amino-acid sequence identity (>80%) [18] and is grouped with At PrR2, which cannot utilize lariciresinol as substrate (Fig. 1 ). Interestingly, in contrast to At PrRs that has substrate preference for pinoresinol, Ii PLR1 from I. indigotica (family Cruciferae, same as A. thaliana ) can reduce both pinoresinol and lariciresinol efficiently with comparable k cat /K m values [18] . The finding that Ii PLR1/ At PrRs, which differ in substrate selectivity, are clustered together suggests that substrate specificity is independent of sequence conservation among PLRs/PrRs. Therefore, the amino-acid residues responsible for PLR/PrR substrate selectivity are difficult to determine merely through sequence analysis, and thus structural information on PLR/PrR enzymes is vital—as are data concerning how these two enzyme types can utilize two different substrates. Fig. 1: Biochemical assays for Ii PLR1 and At PrRs function. a Ii PLR1 efficiently catalyzes the conversion of pinoresinol into lariciresinol and also catalyzes the conversion of lariciresinol into secoisolariciresinol. In contrast, At PrR1/2 exhibit a substrate preference for pinoresinol, yet exhibit only weak activity ( At PrR1) or no activity ( At PrR2) for lariciresinol. b Phylogenetic tree of PLRs/PrRs from different species. c Conversion of pinoresinol into lariciresinol and then into secoisolariciresinol by recombinant Ii PLR1, At PrR1, and At PrR2. The reaction products were analyzed by LC-MS. d Chromatograms for pinoresinol, lariciresinol, and secoisolariciresinol are denoted in black, blue, and red, respectively. Full size image In the present work, we compare crystal structures of Ii PLR1, At PrR1, and At PrR2 and identify residues that may be responsible for the observed substrate selectivity of PLRs and PrRs. Mutagenesis of these residues alters the substrate specificities for pinoresinol and lariciresinol. For example, mutagenesis of Ii PLR1 successfully eliminates the second reaction that converts lariciresinol to secoisolariciresinol, leading to a high accumulation of the pharmaceutically valuable compound lariciresinol. Our study will enable the synthesis of lignans with diverse chemical structures and bioactivities by biotechnological means or by enzyme-assisted chemistry. Characterization of Ii PLR1, At PrR1, and At PrR2 crystal structures To understand both the catalytic mechanism of PLR and the mechanism underlying the substrate specificity of PLRs/PrRs, we chose Ii PLR1, At PrR1, and At PrR2 for a structure study. 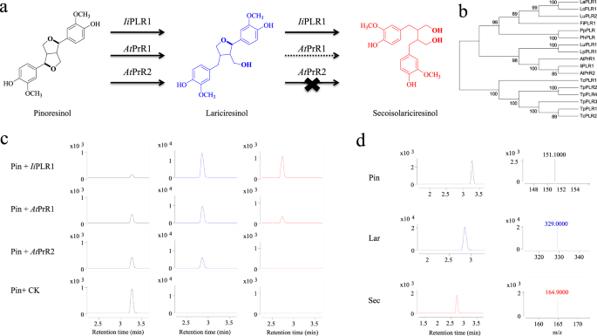Fig. 1: Biochemical assays forIiPLR1 andAtPrRs function. aIiPLR1 efficiently catalyzes the conversion of pinoresinol into lariciresinol and also catalyzes the conversion of lariciresinol into secoisolariciresinol. In contrast,AtPrR1/2 exhibit a substrate preference for pinoresinol, yet exhibit only weak activity (AtPrR1) or no activity (AtPrR2) for lariciresinol.bPhylogenetic tree of PLRs/PrRs from different species.cConversion of pinoresinol into lariciresinol and then into secoisolariciresinol by recombinantIiPLR1,AtPrR1, andAtPrR2. The reaction products were analyzed by LC-MS.dChromatograms for pinoresinol, lariciresinol, and secoisolariciresinol are denoted in black, blue, and red, respectively. The crystal structures were captured in the apo, substrate-bound and/or product-bound forms (Table 1 ). We found that, for all 16 structures we solved, each enzyme adopts a similar head-to-tail dimer conformation (Fig. 2a and Supplementary Fig. 1 ), strongly suggesting that each PLR/PrR functions as a homodimer, consistent with the literature that Tp PLR1 exists as a dimeric entity in solution [17] . Table 1 The crystal structure information of Ii PLR1, At PrR1, and At PrR2 proteins in their apo, NADP + and substrate/product binding forms. Full size table Fig. 2: Structural mechanism of continuous catalytic reactions by Ii PLR1 based on homodimerization. a Dimer formation of Ii PLR1_NAP_ + PIN. Mol-A is shown as cartoon model, with its NBD and SBD colored in light blue and green cyan, respectively. Mol-B is represented as an electrostatic-surface model, on which blue and red colors represent positive and negative charges, respectively. NADP + and (+)-pinoresinol are shown as sticks and colored in orange and yellow, respectively. b Conformational changes were assessed by comparing monomer structures of Ii PLR1_apo (gray) and Ii PLR1_NAP (light orange). The NADP + bound to Ii PLR1_NAP is colored gray. The β4 loops of Ii PLR1_apo and Ii PLR1_NAP are highlighted as purple and green, respectively. c Zoom-in view of the NADPH-binding groove of Ii PLR1_NAP. Residues interacting with NADP + are colored cyan. The conserved GXXGXXG motif is indicated. Residue Val46 involved in dimer formation and substrate binding is shown as a ball-and-stick model and colored magenta. Dotted lines denote possible hydrogen bonds. d Structure comparison of Ii PLR1_NAP_ + PIN and Ii PLR1_NAP. Mol-Bs of Ii PLR1_NAP_ + PIN and Ii PLR1_NAP, Val46s in Ii PLR1_NAP_ + PIN, and Ii PLR1_NAP are colored in marine, orange, magenta, and light yellow, respectively. e Zoom-in view of the substrate-binding groove. Residues of Mol-As in Ii PLR1_NAP_ + PIN and Ii PLR1_NAP are colored green cyan (or light blue) and light yellow, respectively. f Structural comparation of the substrate/product-binding grooves in Ii PLR1_NAP_ + PIN, Ii PLR1_NAP_-LAR (blue white), and Ii PLR1_NAP_-SEC (smudge). The cartoons are generated by PyMOL. g Enzyme assays for wild-type Ii PLR1 and its mutants V46A and V46L. Data are mean±s.d. ( n = 3 independent experiments). Asterisk * indicates significant difference from the wild-type enzyme ( P < 0.05) analyzed by one-way ANOVA with Tukey’s multiple comparisons test. Source data underlying Fig. 2g are provided as a Source Data file. Full size image Taking the structure of Ii PLR1_NAP_+PIN for the purpose of a detailed description, each protomer contains two domains, namely the N-terminal NADPH binding domain (NBD) and the C-terminal substrate binding domain (SBD). The NBD comprises seven β-strands (β1−6, β8) surrounded by six α-helices (α1−5, α7), whereas the SBD comprises two β-strands (β7, β9) with five small α-helices (α6, α8−11). A large groove is formed between NBD and SBD (Fig. 2a ). This groove can be roughly divided into two parts—the positively charged part that associates with the NBD and the hydrophobic part that associates with the SBD. The substrates or products can be clearly defined within the groove (Fig. 2a and Supplementary Fig. 2 ). Several regions (α5 loop, α9-helix, and α9 loop) are partially disordered both in the Ii PLR1_apo and Ii PLR1_NAP structures, for which the differences can be characterized by a RMSD of 0.287 Å, whereas the β4 loop is well defined in the apo structure (Fig. 2b ). Intriguingly, the β4 loop is well defined in the At PrR1_NAP structure but disordered in the At PrR1/2_apo structures (Supplementary Fig. 3 ). These structural differences suggest that the loops are somewhat flexible, and act as a switch to control the binding of NADPH and release of NADP + . Moreover, the β2 loop moves slightly towards NADP + in the Ii PLR1_NAP structure, catering to the entry of the coenzyme (Fig. 2b ). NADP + forms strong hydrogen bonds and hydrophobic interactions with residues within the groove (Fig. 2c ), among which the GXXGXXG motif (considered as the conserved NADPH-binding motif) binds the phosphate and deoxyribose groups, and residues Ala164, Cys165 together with Phe166 fix the position of the catalytically active nicotinamide group. Residue Lys144, which corresponds to the previously reported Lys138 in Tp PLR1 that serves as the general base for catalysis, forms direct hydrogen bonds with NADP + in I i PLR1_apo and Ii PLR1_NAP. Catalytic mechanism of PLR based on its homodimeration The dimers of Ii PLR1_NAP and Ii PLR1_NAP_ + PIN have similar structures, as suggested by a RMSD of 0.362 Å, indeed, even the NADP + moieties could be aligned almost in the same position (Fig. 2d ). Both β4 loops are disordered, further implying their flexibility, but β2 loop and α10-helix from neighboring molecules of Ii PLR1_NAP_ + PIN dimer make contacts with and stabilize the substrate (Fig. 2d, e ). Similar conformational changes of β2 loop and α10-helix can be seen by comparing the structure of At PrR1_NAP_ + PIN with that of At PrR1_NAP and the structure of At PrR2_NAP_ + PIN with that of At PrR2_apo (Supplementary Fig. 4a, b ). (+)-Pinoresinol is inserted as a straight chain deep into the hydrophobic groove, for which the hydrophilic ends are stabilized through the formation of hydrogen bonds with main-chain atoms of Met125 and Gly178, and the hydrophobic region is surrounded by a series of hydrophobic groups (Fig. 2e ). The inner 2-methoxy-phenol group of (+)-pinoresinol forms a sandwich-like π–π stack comprising the nicotinamide head of NADP + and Phe166. Two furan rings in the middle are surrounded by Tyr169 and Phe170 from α6-helix and by His276 and Phe277 from α10-helix. The outer 2-methoxy-phenol group is coordinated by Phe277 and Val46 of β2 loop from a neighboring protomer, which is distant from the NADP + and (+)-pinoresinol of the protomer (Fig. 2 a, c, e ). Further, Lys144 is far away from the furan rings, indicating that it may not participate in catalysis directly. Based on this structure analysis, we propose that both the entry and exit of NADPH are controlled by the β4 loop of Ii PLR1. Once one molecule of (+)-pinoresinol is captured by the narrow hydrophobic groove, each protomer forces the prepositioning of the α10-helix and β2 loop in the other protomer, resulting in tight binding of the substrate. This allows H: transfer from the NADPH to the proximal furan ring of the substrate to produce one molecule of (+)-lariciresinol. Regarding the mechanism of the second catalytic step, we further compared the structures of Ii PLR1_NAP_ + PIN, Ii PLR1_NAP_-LAR and Ii PLR1_NAP_-SEC, which revealed a similar mode for substrate/product binding (Fig. 2f ). Furthermore, Leu46 (corresponding to Val46 in Ii PLR1), His276 and Phe277 of At PrR1 are positioned similar to the corresponding residues of Ii PLR1 to effect substrate binding or product release, except that the β4 loops cover the substrate/product, which are disordered in the Ii PLR1 structures (Fig. 2d and Supplementary Fig. 4a , c, d ). The importance of Val46 for catalysis in Ii PLR1 is underscored by data from a mutational analysis (Fig. 2g ). Mutation of Val46 to Ala improved the conversion of pinoresinol to lariciresinol by ~16%, and the subsequent conversion to secoisolariciresinol was greatly reduced. The Ii PLR1 mutant V46L had little ability to catalyze the conversion of lariciresinol to secoisolariciresinol. These data suggest that Ii PLR1 undergoes substrate-induced conformational changes upon homodimerization to achieve catalysis, and the principle of catalytic reactions using lariciresinol as substrate (second step) appears to be like that using pinoresinol as substrate (first step). Mechanism underlying the substrate selectivity of PLR/PrR A previous study reported that the recombinant At PrR1 can only weakly reduce lariciresinol whereas At PrR2 lacks activity, which is in sharp contrast to all known PLRs [15] . To determine the mechanism underlying this difference in substrate specificity, we confirmed the relative lack of activity for At PrR1/2 (Fig. 1 ) and then carried out a structure analysis of Ii PLR1, At PrR1, and At PrR2. Each of Ii PLR1_NAP_ + PIN/ At PrR1_NAP_ + PIN/ At PrR2_NAP_ + PIN forms a homodimer, and superimposition of the protomers among the three complexes revealed RMSDs of 0.374, 0.365, and 0.308 Å, respectively (Fig. 3 a, c and Supplementary Fig. 1 ). In contrast to Ii PLR1_NAP_ + PIN, the β4 loops of At PrR1_NAP_ + PIN and At PrR2_NAP_ + PIN can be clearly identified (Fig. 3 and Supplementary Fig. 4 ). These well-defined loops twist as an “8” shape and cover both the NADP + -binding and substrate-binding grooves. Within the twisted loop, His93 and His97 “grasp” helices α5 and α10, while Val92 and Phe94 interact directly with (+)-pinoresinol; Arg95 strongly interacts with NADP + as well as each of the GXXGXXG motif and α2-helix from neighboring protomer of the dimer. Similar β4 loops are also observed in all other At PrR1 substrate/product-bound structures, whereas each β4 loop is disordered in the corresponding Ii PLR1 structures, which indicates that the β4 loop may participate in substrate selectivity and, hence, catalysis. Fig. 3: Structural differences among Ii PLR1, At PrR1, and At PrR2 indicating different catalytic capacities. a Structural alignment of dimerized Ii PLR1_NAP_ + PIN (green cyan) and At PrR1_NAP_ + PIN (light gray). b Zoom-in view of dashed box in a . The β4 loop of At PrR1_NAP_ + PIN is highlighted in orange. c Structural alignment of dimerized Ii PLR1_NAP_ + PIN (green cyan) and At PrR2_NAP_ + PIN (slate blue). d Zoom-in view of the dashed box in c . The β4 loop of At PrR2_NAP_ + PIN is highlighted in magenta. For brevity, NADP + and some residues in Ii PLR1 are hidden. The cartoons are generated by PyMOL. Full size image We further explored why the loops behaved differently between Ii PLR1 and the At PrRs. The amino acid sequences of the β4 loops in the three proteins are quite similar (Supplementary Fig. 5 ), but the residue corresponding to Ser98 at the C-terminal end of the loop in Ii PLR1 is replaced as Asn98 in At PrR1/2. Combining the sequence and structural data, the difference can be explained reasonably as follows: the serine side chain is short enough to remain beneath the guanine group of NADPH, whereas the asparagine side chain cannot do so owing to steric hindrance. Consequently, the asparagine lies nearly vertical to the guanine group and points upward in the structure shown in Fig. 3 b, d , and thus the swing of the β4 loop is limited in the At PrR1_NAP structure. As substrate enters the catalytic site, β4 loop can fold and cover the substrate-binding groove (Fig. 3 b, d and Supplementary Figs. 3b and 4a ). Besides the β4 loop, Val46 in Ii PLR1 is replaced with Leu46 in At PrR1, which has the effect of compressing the substrate-binding pocket. Although Val46 is unchanged in At PrR2, the α2-helix and β2 loop from the neighboring protomer move closer to the substrate upon its entry at the catalytic site, further condensing the pocket. The relative movement of dimers between At PrR2 and Ii PLR1 (as suggested by the ~9° shift shown in Fig. 3c ) could be induced by different dimer orientations. Two molecules of the dimer exhibit relative torsion in At PrR2, and consequently, Val46 is forced deeper into the substrate-binding pocket compared with what occurs in Ii PLR1. Therefore, the entrance and orientation of the substrate in At PrR1/2 is more tightly controlled than in Ii PLR1. Mutagenesis-based alteration of the substrate selectivity Based on the structural analysis of Ii PLR1, At PrR1 and At PrR2, the importance of the candidate amino acids controlling substrate specificity was verified through site-directed mutagenesis. Enzymatic assays using pinoresinol as substrate revealed that the Ii PLR1 mutations including V46A, V46L, S98A, S98H, and S98N somewhat enhanced the conversion rate of lariciresinol while significantly reduced that of secoisolariciresinol, and mutants V46A, S98A, and S98H had > 40% conversion rates for lariciresinol (Fig. 4a ), suggesting that residues 46 and 98 are critical for the substrate preference. 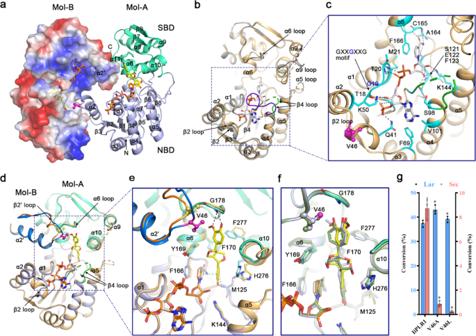Fig. 2: Structural mechanism of continuous catalytic reactions byIiPLR1 based on homodimerization. aDimer formation ofIiPLR1_NAP_ + PIN. Mol-A is shown as cartoon model, with its NBD and SBD colored in light blue and green cyan, respectively. Mol-B is represented as an electrostatic-surface model, on which blue and red colors represent positive and negative charges, respectively. NADP+and (+)-pinoresinol are shown as sticks and colored in orange and yellow, respectively.bConformational changes were assessed by comparing monomer structures ofIiPLR1_apo (gray) andIiPLR1_NAP (light orange). The NADP+bound toIiPLR1_NAP is colored gray. The β4 loops ofIiPLR1_apo andIiPLR1_NAP are highlighted as purple and green, respectively.cZoom-in view of the NADPH-binding groove ofIiPLR1_NAP. Residues interacting with NADP+are colored cyan. The conserved GXXGXXG motif is indicated. Residue Val46 involved in dimer formation and substrate binding is shown as a ball-and-stick model and colored magenta. Dotted lines denote possible hydrogen bonds.dStructure comparison ofIiPLR1_NAP_ + PIN andIiPLR1_NAP. Mol-Bs ofIiPLR1_NAP_ + PIN andIiPLR1_NAP, Val46s inIiPLR1_NAP_ + PIN, andIiPLR1_NAP are colored in marine, orange, magenta, and light yellow, respectively.eZoom-in view of the substrate-binding groove. Residues of Mol-As inIiPLR1_NAP_ + PIN andIiPLR1_NAP are colored green cyan (or light blue) and light yellow, respectively.fStructural comparation of the substrate/product-binding grooves inIiPLR1_NAP_ + PIN,IiPLR1_NAP_-LAR (blue white), andIiPLR1_NAP_-SEC (smudge). The cartoons are generated by PyMOL.gEnzyme assays for wild-typeIiPLR1 and its mutants V46A and V46L. Data are mean±s.d. (n= 3 independent experiments). Asterisk * indicates significant difference from the wild-type enzyme (P< 0.05) analyzed by one-way ANOVA with Tukey’s multiple comparisons test. Source data underlying Fig.2gare provided as a Source Data file. Taking V46A as an example for the kinetic analysis, its K m value for pinoresinol (29.4 ± 1.62 μM) is comparable with that for lariciresinol (26.5 ± 0.60 μM), however its V max for pinoresinol (3.22 ± 0.68 μM min −1 ) is 140-fold higher than that for lariciresinol (0.023 ± 0.0013 μM min −1 ), and its k cat /K m for pinoresinol (3.88 ± 0.65 μM −1 min −1 ) is 126-fold higher than that for lariciresinol (0.031 ± 0.002 μM −1 min −1 ) (Table 2 ). Compared with wild-type Ii PLR1 [18] , the activity of mutant V46A towards pinoresinol increases 4-fold, whereas that towards lariciresinol decreases 98% with regard to k cat /K m values. These results indicate mutant V46A enhances catalytic efficiency for the first reaction but dramatically eliminates the second reaction. Consistent with the data for Ii PLR1, At PrR1 mutants L46A and L46V could enhance the conversion rate of lariciresinol and partially reduce that of secoisolariciresinol (Fig. 4a ), which confirmed the importance of these two sites in substrate binding and product release thus in catalysis. As expected, mutants N98A and N98S in At PrR1 had increased activity for secoisolariciresinol production compared with wild type (Fig. 4a ), strongly implying that residue 98 controls the swing of the β4 loop, which affects substrate binding and catalysis. Interestingly, At PrR2 mutant N98S could utilize lariciresinol to produce secoisolariciresinol, with a conversion rate of 1.91%, in contrast to the wild type which lacks this activity (Fig. 4a ). Other At PrR2 mutants, including V46A, V46L, and N98A, varied in their activities for pinoresinol, as indicated by the relative rates of conversion to lariciresinol (Fig. 4a ). Similar results were obtained for conversion of lariciresinol to secoisolariciresinol (Fig. 4b ). Altogether, the structure-guided mutagenesis indeed could switch the substrate specificity of PLR/PrR, e.g., the Ii PLR1 mutant V46A had increased preference for pinoresinol but little catalytic activity for lariciresinol, whereas the At PrR2 mutant N98S gained the activity to catalyze the conversion of lariciresinol to secoisolariciresinol (Fig. 4c ). Fig. 4: Percent conversion of pinoresinol to lariciresinol and subsequently to secoisolariciresinol by mutants of Ii PLR1, At PrR1 and At PrR2. a Conversion of pinoresinol into lariciresinol and subsequently to secoisolariciresinol. b Conversion of lariciresinol into secoisolariciresinol. Data are mean ± s.d. ( n = 3 independent experiments). Asterisk (*) indicates significant difference from the wild-type enzyme ( P < 0.05) analyzed by one-way ANOVA with Tukey’s multiple comparisons test. Source data underlying Fig. 4a, b are provided as a Source Data file. c LC-MS determination of the products as catalyzed by Ii PLR1, Ii PLR1_V46A, At PrR2 and At PrR2_N98S. Full size image Table 2 Kinetic properties of Ii PLR1_V46A. Full size table Taking structure and enzymology data together, we proposed a three-step catalytic mechanism for PLR based on its homodimerization. First, the protomers of dimeric PLRs recruit free NADPH through the very flexible β4 loop. Second, pinoresinol binds into one protomer via the substrate-binding groove, and the other protomer of the homodimer helps stabilize the substrate. Subsequently, pinoresinol receives H: from NADPH and be reduced to lariciresinol released later. Third, free lariciresinol is bound by another reductive PLR molecule and fixed by another homodimer, and then the lariciresinol is reduced to secoisolariciresinol and finally released (Fig. 5 and Supplementary Movie 1 ). Fig. 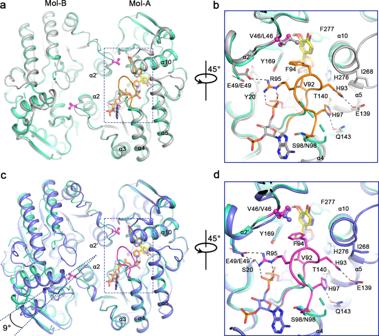Fig. 3: Structural differences amongIiPLR1,AtPrR1, andAtPrR2 indicating different catalytic capacities. aStructural alignment of dimerizedIiPLR1_NAP_ + PIN (green cyan) andAtPrR1_NAP_ + PIN (light gray).bZoom-in view of dashed box ina. The β4 loop ofAtPrR1_NAP_ + PIN is highlighted in orange.cStructural alignment of dimerizedIiPLR1_NAP_ + PIN (green cyan) andAtPrR2_NAP_ + PIN (slate blue).dZoom-in view of the dashed box inc. The β4 loop ofAtPrR2_NAP_ + PIN is highlighted in magenta. For brevity, NADP+and some residues inIiPLR1 are hidden. The cartoons are generated by PyMOL. 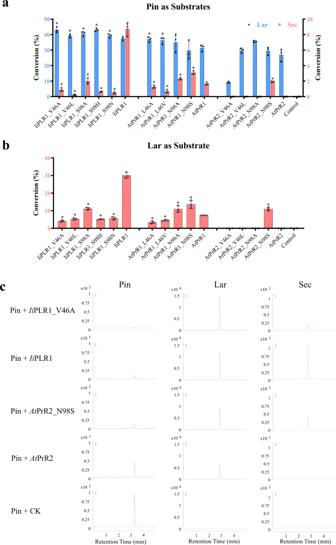Fig. 4: Percent conversion of pinoresinol to lariciresinol and subsequently to secoisolariciresinol by mutants ofIiPLR1,AtPrR1 andAtPrR2. aConversion of pinoresinol into lariciresinol and subsequently to secoisolariciresinol.bConversion of lariciresinol into secoisolariciresinol. Data are mean ± s.d. (n= 3 independent experiments). Asterisk (*) indicates significant difference from the wild-type enzyme (P< 0.05) analyzed by one-way ANOVA with Tukey’s multiple comparisons test. Source data underlying Fig.4a, bare provided as a Source Data file.cLC-MS determination of the products as catalyzed byIiPLR1,IiPLR1_V46A,AtPrR2 andAtPrR2_N98S. 5: Model depicting the catalytic processes of PLRs and PrRs. The blue dumbbell-shaped objects represent switches composed of β4 loops. A movie showing how the enzymes change conformation throughout a single round of catalysis can be found in Supplementary Movie 1 . Full size image Importantly, the PrRs have more strict requirements for the binding and orientation of lariciresinol compared with PLRs, so PrRs cannot efficiently carry out the third step (Fig. 5 ). Hence, the substrate-specificity mechanism of PLRs/PrRs could be that residues located around the substrate-binding pocket and within the loop, together with residues that promote homodimerization, form the appropriate hydrophobic environment for binding a specific substrate. Mutation increases lariciresinol and reduces secoisolariciresinol production in vivo Enzymatic assays indicated that certain Ii PLR1 mutants had increased activity for producing lariciresinol from pinoresinol in vitro (Fig. 4 ). Therefore, these Ii PLR1 mutant genes were selected for lariciresinol production using pinoresinol-producing E. coli [19] . Because matairesinol, which is derived from secoisolariciresinol, is detectable only when CueO (multicopper oxidase), PLR and SDH (secoisolariciresinol dehydrogenase) are individually expressed in cells [20] , each of wild-type Ii PLR1 and its mutants were co-cultured in pinoresinol-producing E. coli [19] . 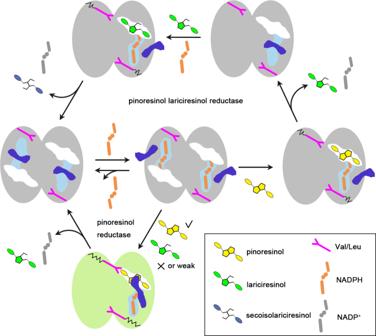Fig. 5: Model depicting the catalytic processes of PLRs and PrRs. The blue dumbbell-shaped objects represent switches composed of β4 loops. A movie showing how the enzymes change conformation throughout a single round of catalysis can be found in Supplementary Movie1. 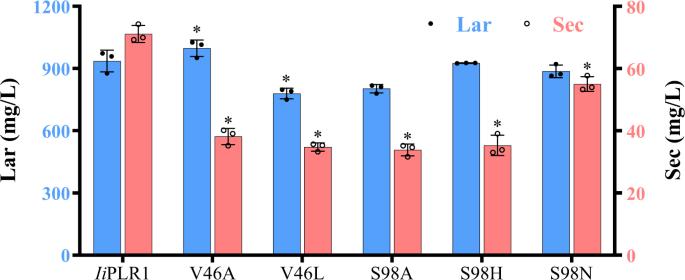Fig. 6: Lariciresinol production through co-culture of different strains harboring a plasmid encodingIiPLR1 or its single-site mutants with pinoresinol-producing cells. Data are mean±s.d. (n= 3 independent experiments). Asterisk (*) indicates significant difference from the wild-type enzyme (P< 0.05) analyzed by one-way ANOVA with Tukey’s multiple comparisons test. Source data are provided as a Source Data file. Consistent with the enzyme assay results, Ii PLR1_V46A produced the greatest amount of lariciresinol (997.79 mg L −1 compared with 936.14 mg L −1 for wild-type). However, mutants V46L, S98A, S98H, and S98N were not as efficient as wild-type cells at producing lariciresinol, which was opposite to the results from in vitro enzyme assays. This may reflect the potential effects of complex metabolic networks and feedback mechanisms in vivo, which are not relevant to in vitro enzyme assays. Moreover, the provision of NADPH is tightly regulated in prokaryotic systems, which also may influence the activity of PLRs. Notably, all the Ii PLR mutants produced significantly less secoisolariciresinol than wild-type cells, i.e., by 22.7–52.5%; in particular, Ii PLR_V46A produced 46.4% less secoisolariciresinol than wild type (Fig. 6 ). These results paralleled those obtained in vitro with the Ii PLR1 mutants in which there was elimination of the second catalytic step, i.e., the conversion of lariciresinol to secoisolariciresinol (Fig. 4 ). Taken together, our results establish a promising route for the production of lariciresinol by synthetic biology strategies, and mutant Ii PLR_V46A mutant would be a good candidate for use in the large-scale production of the pharmaceutically valuable compound lariciresinol. Fig. 6: Lariciresinol production through co-culture of different strains harboring a plasmid encoding Ii PLR1 or its single-site mutants with pinoresinol-producing cells. Data are mean±s.d. ( n = 3 independent experiments). Asterisk (*) indicates significant difference from the wild-type enzyme ( P < 0.05) analyzed by one-way ANOVA with Tukey’s multiple comparisons test. Source data are provided as a Source Data file. Full size image The molecular mechanism of substrate selectivity of PLR/PrR has attracted particular interest owing to the key role of these enzymes in lignan biosynthesis. However, the lack of structural results—especially for PLRs/PrRs in complex with different substrates—has limited our understanding of the mechanism underlying enzyme specificity. In the present study, we characterized crystal structures of Ii PLR1, At PrR1, and At PrR2 in complex with their various substrates. Several residues participating in substrate binding and catalysis were identified either directly or indirectly based on structural analysis, and these residues were validated by enzyme assays. All these data provide solid evidence to explore the mechanistic basis of substrate selectivity for PLRs/PrRs. Besides residues 46 and 98 in Ii PLR1 and At PrRs that we identified as being critical for binding and catalysis, residues Phe166, Tyr169, Phe170, His276, and Phe277 within the substrate-binding groove were also strongly correlated with enhanced substrate binding and catalysis. We further deduced that any residue in PLRs/PrRs around the hydrophobic groove or affecting homodimerization may impact the conformation of the active site, thereby dictating substrate selectivity (Supplementary Figs. 5 and 6 ). Consequently, it is not difficult to understand why mutant L174I of C. sinensis PLR1 can hardly reduce pinoresinol and specifically catalyze the conversion of lariciresinol to secoisolariciresinol [16] , i.e., because Leu174 points directly toward Tyr163 and thus may indirectly promote substrate recognition. In addition, PLRs also display substrate stereochemical selectivity, which contributes to the enantiomeric diversity of lignans [21] , [22] , [23] , [24] . We found this to be true for Ii PLR1, which gave comparable k cat / K m values for both (±)-pinoresinol and (±)-lariciresinol in the range of 0.9–1.6 µM −1 min −1 , although no experiments with respect to the enantio-specificity of this enzyme have been performed [12] , [18] . Despite past research on this topic, however, the mechanism underlying the substrate stereochemical selectivity of PLRs remains unclear. Comparison of the enantiospecifically opposite PLRs Tp PLR1 and Tp PLR2 suggests that F164, V268, and L272 in Tp PLR1 contribute to the catalysis of (−)-pinoresinol, whereas L164, G268, and F272 in Tp PLR2 prefer to bind (+)-pinoresinol [17] . Nevertheless, site-directed mutagenesis carried out in flax indicates that these positions are insufficient to determine enantiospecificity [21] . Based on amino-acid sequence and structural analyses, it seems that residues Phe94 and Phe277 in Ii PLR1/ At PrR1 may act in concert to determine the enantiospecificity of PLRs (Supplementary Fig. 6 ). These two residues are highly conserved in PLRs that have no enantio-specificity, whereas Ile94 and Tyr277 are present in PLRs that have a strict substrate preference for (+)-pinoresinol. Moreover, in Linum usitatissimum PLR1 ( Lu PLR1), which has strict enantiospecificity for (–)-pinoresinol, a leucine residue is deleted as are two other residues on β4 loop (corresponding to the β4 loop of Ii PLR1, where Phe94 is located). Unfortunately, we could not obtain sufficient amounts of the enantiomerically pure substrates to carry out the experiments necessary to establish the enantio-selectivity. Nature uses a dazzling array of enzymes to produce diverse natural products. However, some modifications are challenging to control because the relative lack of substrate specificity often generates undesired byproducts. Ii PLR1 plays an important role in the biotechnological production of lariciresinol [18] , which represents the most important component for the antibacterial, antiviral, and the immune-regulatory effects of the traditional Chinese medicine Radix Isatidis [3] , [25] , [26] . The fact that Ii PLR1 can efficiently utilize both pinoresinol and lariciresinol as substrates [18] suggests that the biosynthetic efficiency towards the pharmaceutically valuable compound lariciresinol in Radix Isatidis has been hampered by the relatively low substrate specificity of Ii PLR1. In our present work, structure-guided mutagenesis successfully switched the substrate specificity of Ii PLR1, leading to overproduction of lariciresinol and reduced production of secoisolariciresinol by E. coli . Our study provides insight into the molecular mechanism underlying the substrate specificity of PLRs/PrRs, and paves the way for the manufacture of lariciresinol through microbial fermentation. Moreover, this work suggests the possibility of using targeted mutagenesis of Ii PLR to improve the efficiency of synthesizing bioactive compounds in I. indigotica using gene-editing technologies [27] , [28] . Phylogenic analysis of plant PLRs Phylogenetic relationships were analyzed using the maximum likelihood method with the pairwise deletion option in MEGA 6.06. Tree reliability was estimated using a bootstrap analysis of 1000 replicates [29] . Plant PLR amino-acid sequences used in the phylogenic analysis were retrieved from GenBank, including Tp PLR1 (AAF63507.1), Tp PLR2 (AAF63508.1), Tp PLR3 (AAF63509.1), Tp PLR4 (AAF63510.1), Pp PLR (AHL21381.1), La PLR1 (CAH60857.1), Lu PLR1 (CAH60858.1), Lu PLR2 (ABW24501.1), Lp PLR1 (ABM68630.1), Lc PLR1 (ABW86959.1), Ph PLR (ACF71492.1), Tc PLR1 (AZL88516.1), Tc PLR2 (AZL88517.1), Fi PLR1 (AAC49608.1), Ii PLR1(AEA42007.1), At PrR1 (NP_174490.1), and At PrR2 (NP_193102.1). Heterologous expression of Ii PLR1, At PrR1, and At PrR2 in E. coli Total RNA was extracted from leaves of wild-type I. indigotica or A. thaliana using TRIzol Reagent (GIBCO BRL). The mRNA was reverse transcribed with oligo dT to generate cDNA as a template for PCR. Full-length cDNA sequences of Ii PLR1 (GenBank accession no. JF264893), At PrR1 (AY065214) and At PrR2 (BT002882) were cloned into pET-duet-1 (Novagen, USA) to generate Ii PLR1-pET, At PrR1-pET, and At PrR2-pET, respectively. The primers used are listed in Supplementary Table 1 . E. coli Rosetta (DE3) cells were transformed with purified plasmid DNA and then grown at 37 °C to an OD 600 of 0.8. Then, protein expression was induced by adding 0.5 mM isopropyl β- d -thiogalactoside (IPTG, final concentration) with incubation overnight at 16 °C. Cells were collected, resuspended in buffer A (20 mM Tris-HCl pH 8.0, 100 mM NaCl), and lysed with a French press. The lysate was centrifuged at 20,000× g for 45 min, and the supernatant was applied to a Ni-NTA column equilibrated with buffer A supplemented with 25 mM imidazole. Bound protein was eluted using buffer A containing 250 mM imidazole and was concentrated for further purification on a Superdex-200 column equilibrated with buffer A. Protein purity was assessed by SDS-PAGE (12% polyacrylamide), and protein concentration was determined by the Bradford method [30] . Crystallization, data collection, and structure determination The full-length Ii PLR1/ At PrR1/ At PrR2 were purified as described above and concentrated to 5–10 mg mL −1 for crystallization. Aliquots of each concentrated protein sample were mixed 1:1 with reservoir solution, and crystals were grown at 20 or 4 °C in one week using the sitting-drop vapor-diffusion method. For co-crystals, protein was combined with NADP + at a 1:5 molar ratio, and protein with NADP + and substrate/product at a 1:5:10 molar ratio. For reservoir solutions, Ii PLR1 apo and co-crystals were grown with 0.2 M sodium citrate tribasic, 0.1 M sodium citrate/citric acid, pH 4.0 and 20% polyethylene glycol (PEG) 3350; At PrR1 apo crystals were grown in 0.2 M lithium chloride, 20% w/v PEG 3350; At PrR1_NAP, At PrR1_NAP_ + PIN, At PrR1_NAP_ + LAR and At PrR1_NAP_-SEC were grown in 0.2 M sodium fluoride, 20% w/v PEG 3350; At PrR1_NAP_-PIN and At PrR1_NAP_-LAR crystals were grown in 0.2 M sodium malonate, pH 6.0, 20% w/v PEG 3350; At PrR2 apo crystals were grown in 0.2 M magnesium chloride, 0.1 M sodium HEPES, pH 7.5 and 25% PEG 3350; At PrR2_NAP_ + PIN crystals were grown in 2.1 M DL malic acid, pH 7.0. The crystals were cryoprotected by serial transfers into reservoir solutions supplemented with 30% (v/v) glycerol and then flash-cooled in liquid nitrogen. Data collections were performed at the BL17U1 and BL19U1 beamline of the Shanghai Synchrotron Radiation Facility. The data were processed with HKL3000 [31] , and the initial phase was determined by molecular replacement with Phenix [32] using the crystal structure of Tp PLR1 (PDB ID: 1QYD [ https://doi.org/10.2210/pdb1qyd/pdb ]) as a template. The structure models were firstly auto-built in Coot [33] and then refined by iterative rounds of manual adjustment with Coot and refinement with Phenix. The statistics of data collection and structure refinement are shown in Supplementary Tables 2 – 5 . Site-directed mutagenesis of Ii PLR1, At PrR1, and At PrR2 and enzymatic assays Single-site mutagenesis was achieved through one-step PCR, and mutants were verified with Sanger sequencing. All primers are listed in Supplementary Table 1 . After expression and purification of recombinant enzymes under the aforementioned conditions, the results for the enzyme assays for mutants were compared with those for wild-type recombinant Ii PLR1, At PrR1, and At PrR2 as follows. Enzyme activity assays were conducted strictly according to our previous work [18] . Assay mixtures (1 mL) consisted of TG buffer (50 mM Tris-HCl, 10% [w/v] glycerol, pH 7.0), 150 μM NADPH], 100 μM pinoresinol, or 100 μM lariciresinol and 5 μg of purified protein. Assays without a fusion protein were used as controls. Protein, buffer, and substrate were pre-incubated for 5 min at 30 °C, and each reaction was initiated by addition of NADPH and terminated after 30 min by addition of 300 μL ethyl acetate. Each assay mixture was extracted with ethyl acetate (3 × 300 μL total). The combined ethyl acetate phases were dried under vacuum, and the residue was dissolved in 1 mL methanol. Conversion rate was then determined. The content of pinoresinol, lariciresinol and secoisolariciresinol was determined by LC-MS using a triple-quadrupole mass spectrometer (Model 6410, Agilent, Santa Clara, CA) following our published methods [18] . MassHunter Qualitative Analysis B.06.00 was used for the data analysis. The selected transitions of m / z were 357 → 151 for pinoresinol, 359 → 329 for lariciresinol, and 361 → 164 for secoisolariciresinol. All standards were purchased from Sigma-Aldrich (St. Louis, MO). For determination of V max and K m values for Ii PLR1_V46A, 10 different concentrations of substrate (pinoresinol or lariciresinol; 5–200 μM) and 1 μg purified protein were used. Samples were incubated at 30 °C for 5 min (during which substrate consumption was ≤10%). Samples without protein were used as controls. The rate of substrate consumption was calculated for kinetic analysis. V max and K m values were determined from Lineweaver-Burk plots, and k cat was determined by dividing V max by the enzyme concentration. Bioconversion For the production of lariciresinol, biotransformation was divided into two modules, namely the accumulation and conversion of the precursor, pinoresinol. E. coli strain strOpr2 carrying plasmid pET28a-Prx02-PsVAO was used to produce pinoresinol [19] , whereas E. coli BL21(DE3) carrying a plasmid encoding Ii PLR1 or its mutants was used for conversion of pinoresinol to lariciresinol. These E. coli strains were cultured in LB medium at 37 °C with shaking (220 rpm) for 12 h as seed cultures, and then a 2% seed culture was transferred to a 250-mL shaker flask containing 25 mL TB medium. After culturing for 2–2.5 h at 37 °C and 220 rpm, 500 μM IPTG (final concentration) was added to the medium with continued cultivation for 12 h at 25 °C and 220 rpm. These cells were used for pinoresionol accumulation and conversion, respectively. Cells from E. coli strain strOpr2 were harvested by centrifugation at 4 °C and 3724× g for 30 min and then resuspended in phosphate-buffered saline (pH 7.0) to adjust the OD 600 value to 20. Then 0.15% (v/v) eugenol was added into 15 mL of the resuspension at 0, 1, 3, 5, and 7 h for pinoresinol accumulation (20 °C, 220 rpm). At 9 h, 15 ml of a culture of E. coli expressing Ii PLR1 and each mutant (OD 600 = 20) was added to determine the conversion of pinoresinol to lariciresinol (25 °C, 220 rpm), and samples were taken after 20 h. The concentration of each of lariciresinol and secoisolariciresinol was determined by HPLC. Statistical analysis All the experiments in this paper were repeated at least three times and results from representative data sets are presented. GraphPad Prism (version 9.1.0) was used for the statistical analysis. The statistical evaluations used one-way analysis of variance (ANOVA) with multiple comparisons, followed by Tukey tests. The results were considered statistically significant at * P < 0.05. Further information on research design is available in the Nature Research Reporting Summary linked to this article.